Using synthetic templates to design an unbiased multiplex PCR assay T and B cell receptor loci undergo combinatorial rearrangement, generating a diverse immune receptor repertoire, which is vital for recognition of potential antigens. Here we use a multiplex PCR with a mixture of primers targeting the rearranged variable and joining segments to capture receptor diversity. Differential hybridization kinetics can introduce significant amplification biases that alter the composition of sequence libraries prepared by multiplex PCR. Using a synthetic immune receptor repertoire, we identify and minimize such biases and computationally remove residual bias after sequencing. We apply this method to a multiplex T cell receptor gamma sequencing assay. To demonstrate accuracy in a biological setting, we apply the method to monitor minimal residual disease in acute lymphoblastic leukaemia patients. A similar methodology can be extended to any adaptive immune locus. The genomes of B and T cells undergo combinatorial shuffling (that is, somatic rearrangement) of cell-surface receptor gene segments, allowing for a finite genome to encode many trillions of possible receptors. Most of the diversity in these B-cell receptors and T-cell receptors (TCRs) is contained in the complementary determining region 3 (CDR3) regions of the heterodimeric cell-surface receptors. For the TCR, the CDR3 regions are formed by rearrangements of variable and joining (VJ) gene segments for the α and γ chains and variable, diversity and joining (VDJ) gene segments for the β and δ chains. The V-J, V-D and D-J junctions are imperfect rearrangements, and can have both deletions and non-templated nucleotide insertions [1] . These mechanisms create the large diversity of clonal B-cell receptors and TCRs within a healthy person, which is sufficient for one or more adaptive immune cells to bind to almost any antigen and initiate an immune response [2] , [3] . In addition to the generation of a diverse set of antigen receptor molecules, the adaptive immune system functions in part by clonal expansion; in an adult human, there are millions of different TCR rearrangements carried by several billion circulating T-cells [4] , [5] , [6] , [7] . Accurately measuring changes in the abundance of each clone is vital for understanding the dynamics of an adaptive immune response. We have developed a multiplex PCR and sequencing approach to monitor the human adaptive immune repertoire [4] , [8] and comprehensively assess its diversity. The different V and J gene segments do not share nucleotide sequence of sufficient length to design a common primer to amplify all combinations. The closest shared sequences to the CDR3 regions are thousands of bases up or down stream of introns. Multiplex PCR is an efficient method for amplifying multiple loci simultaneously. However, multiplex PCR poses unique challenges because all primers must function under the same reaction conditions, which should not only allow each primer to anneal to its true target sequence, but minimize non-specific amplification and avoid production of primer-dimers. Small variations in annealing kinetics can have a large impact on primer amplification efficiency, producing biased PCR product libraries where the observed frequency of each amplicon is not proportional to the original frequency of the input template. In extreme cases, such bias can result in undetectable levels of specific under-amplifying target templates. A bias-free assay is critical for studies aiming to quantitatively measure the frequency of specific immune receptor rearrangements, such as minimal residual disease (MRD) monitoring in leukaemia [9] , [10] , [11] , [12] , following exposure-specific immune repertoires over time [13] , [14] and research to study basic B- and T-cell biology [15] , [16] . To address this issue, we develop a synthetic analogue of a somatically rearranged immune receptor locus (human TCRG ) to quantify and correct multiplex PCR amplification bias. As the actual in vivo TCRG repertoire is a priori impossible to know, we generated a synthetic repertoire that includes a template for every possible V/J combination. Using these synthetic templates, we identify and correct the amplification bias present in our initial assay. We first measure the precise composition of our reference template pool before and after amplification. We then measure the effect of primer concentration on amplification rates, and use these data to titre the relative concentration of each primer in the multiplex reaction such that all V/J combinations amplified with similar efficiencies. Residual differences in amplification efficiency are removed computationally using experimentally derived normalization factors. Finally, we demonstrate a clinical application for the quantitative measurement of clonal TCRG sequences in the context of MRD monitoring of T-cell acute lymphoblastic leukaemia (T-ALL) patients. Synthesis of immune receptor templates We construct a set of synthetic TCRG reference sequence templates to represent the complex nature of somatically rearranged immune receptor targets. To address amplification bias due to differential primer usage in our multiplex PCR, we design one template for each combination of V and J gene segments; we synthesize 56 synthetic templates of 495 bp, as shown in Fig. 1 . The 56 templates represent all possible pairs between 14 V segments and 4 J segments. (J segments 1 and 2 are sequence identical within our target region and were treated as one sequence.). All 56 synthetic molecules are combined into a single, equimolar template pool. To confirm the precise frequency of each individual template in the pool, we use primers coupling the universal primer sequences UA and UB at the 5′- and 3′-ends of the templates and perform sequencing-by-synthesis (Illumina platform). To screen out low-level synthesis errors, only sequences perfectly matching the expected template sequence are considered for all calculations. We show, by replication and by altering the number of PCR cycles, that this process does not introduce detectable amplification bias ( Fig. 2 ). Sequencing allows us to determine the precise relative proportion of each of the synthetic immune receptors in our target pool and thus use it as a validated input for testing our TCRG primer mixtures. 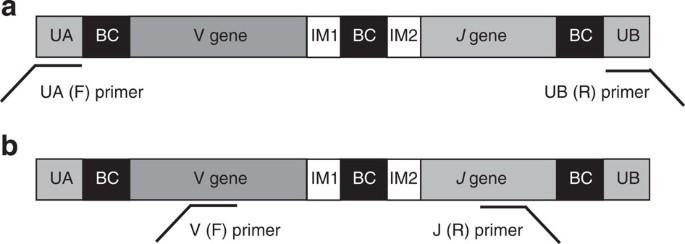Figure 1: Synthetic template design and quantification. Synthetic templates include from left to right, a universal primer (UA), a 16-bp template-specific barcode (BC), 300 bp of aTCRGV gene (Vgene), a 9-bp synthetic template internal marker (IM1), a repeat of the barcode, a 9-bp synthetic template internal marker (IM2), 100 bp of aTCRG Jgene (J gene), a third repeat of the barcode, and a reverse universal primer (UB). The entire template is 495 bp long. (a) We use sequencing to characterize a pool of 56 synthetic templates. Illumina adaptors are first added to the templates by low-cycle PCR. PCR primers contain universal primers on the 3′-end and Illumina sequencing adaptors on the 5′-end. These Illumina tailed synthetic templates are then sequenced using a UB primer. The third barcode is used to identify the frequency of each template in the pool. (b) The characterized pool of syntheticTCRGtemplates is used to assess PCR amplification bias. The VF and JR multiplex PCR primers contained the gene specific sequences on the 3′-end and universal adaptor sequences on the 5′-end. Low-cycle PCR is used to integrate Illumina sequencing adaptors and the resultant amplicon is sequenced on the Illumina MiSeq using JR sequencing primers and the second internal barcode is used to precisely identify each template. Figure 1: Synthetic template design and quantification. Synthetic templates include from left to right, a universal primer (UA), a 16-bp template-specific barcode (BC), 300 bp of a TCRG V gene ( V gene), a 9-bp synthetic template internal marker (IM1), a repeat of the barcode, a 9-bp synthetic template internal marker (IM2), 100 bp of a TCRG J gene (J gene), a third repeat of the barcode, and a reverse universal primer (UB). The entire template is 495 bp long. ( a ) We use sequencing to characterize a pool of 56 synthetic templates. Illumina adaptors are first added to the templates by low-cycle PCR. PCR primers contain universal primers on the 3′-end and Illumina sequencing adaptors on the 5′-end. These Illumina tailed synthetic templates are then sequenced using a UB primer. The third barcode is used to identify the frequency of each template in the pool. ( b ) The characterized pool of synthetic TCRG templates is used to assess PCR amplification bias. The VF and JR multiplex PCR primers contained the gene specific sequences on the 3′-end and universal adaptor sequences on the 5′-end. Low-cycle PCR is used to integrate Illumina sequencing adaptors and the resultant amplicon is sequenced on the Illumina MiSeq using JR sequencing primers and the second internal barcode is used to precisely identify each template. 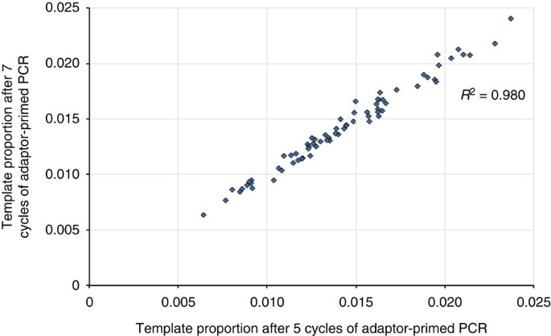Figure 2: Measurement stability of the template pool after amplification by adaptor-primed PCR. To validate our ability to quantify the synthesizedTCRGtemplate pool by low-cycle PCR amplification using universal adaptors, we compare data from five cycles of PCR (including two cycles of exponential growth) and seven cycles of PCR (including four cycles of exponential growth). The proportional representation of each template in these two reactions is graphed above. The excellent agreement we see between these two PCR experiments gives us high confidence that adaptor-primed PCR is essentially unbiased and allows us to accurately assay the relative concentration of each target template in the template pool. Full size image Figure 2: Measurement stability of the template pool after amplification by adaptor-primed PCR. To validate our ability to quantify the synthesized TCRG template pool by low-cycle PCR amplification using universal adaptors, we compare data from five cycles of PCR (including two cycles of exponential growth) and seven cycles of PCR (including four cycles of exponential growth). The proportional representation of each template in these two reactions is graphed above. The excellent agreement we see between these two PCR experiments gives us high confidence that adaptor-primed PCR is essentially unbiased and allows us to accurately assay the relative concentration of each target template in the template pool. Full size image Identifying amplification bias We design 10 forward primers that anneal to the 14 known V segments (VF), and 4 reverse primers that anneal to the 5 J segments (JR) to amplify across rearranged CDR3 regions ( Table 1 ). Primers are designed to be T m -matched and to yield similar product lengths for all V–J pairings; we anticipate that these primers could amplify all possible CDR3 rearrangements at the locus, albeit with unknown amplification bias. Primers are also placed so as to avoid spanning known alleles of the V and J segments, and therefore primer annealing kinetics should be identical for all known alleles of any specific V or J segment. Table 1 Primer Sequences. Full size table To identify off-target amplification, we amplify the TCRG synthetic template pool with only one VF primer at a time multiplexed with all JR primers (or vice versa). These primer specificity tests show that five of the VF primers ( TCRGV01, V02-3-4-5-8, V05P, V06, V07 ) amplify the same family of TCRGV gene segments ( Fig. 3 ). Using these data, we reduce the number of VF primers by four (keeping only the primer designed against V02-3-4-5-8 for all of the V segments above), and only continue with six specific V gene primers. All other VF and JR primers show high, but not complete specificity ( Fig. 3 ), for the expected TCRG target templates. 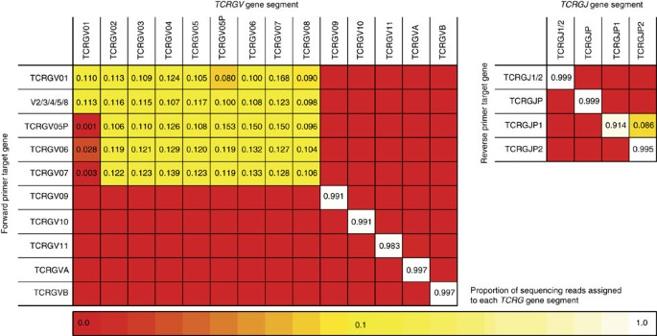Figure 3:TCRGVF and JR primer specificity experiments. We prepare 10 mixtures containing a single VF primer combined with all JR primers, and four mixtures containing a single JR primer combined with all VF primers. We then amplify ourTCRGsynthetic template pool with each of these mixtures and determine the proportion of sequence reads that corresponded to each of theTCRGgene segments: top left, results from the 10 VF primers, targeting 14TCRGVgene segments; top right, results from the four JR primers target fiveTCRGJgene segments. Overall, individual VF and JR show high specificity for their intended targets with the exception of five VF primers that each have extensive cross-priming for the same group of nineTCRGVgene segments. Based on these results, we remove four of these five primers from the assay, resulting in the targeting of nineTCRGVgene segments by a single primer (the VF primer originally targeting V02, V03, V04, V05 and V08). Figure 3: TCRG VF and JR primer specificity experiments. We prepare 10 mixtures containing a single VF primer combined with all JR primers, and four mixtures containing a single JR primer combined with all VF primers. We then amplify our TCRG synthetic template pool with each of these mixtures and determine the proportion of sequence reads that corresponded to each of the TCRG gene segments: top left, results from the 10 VF primers, targeting 14 TCRGV gene segments; top right, results from the four JR primers target five TCRGJ gene segments. Overall, individual VF and JR show high specificity for their intended targets with the exception of five VF primers that each have extensive cross-priming for the same group of nine TCRGV gene segments. Based on these results, we remove four of these five primers from the assay, resulting in the targeting of nine TCRGV gene segments by a single primer (the VF primer originally targeting V02, V03, V04, V05 and V08). Full size image To identify the overall baseline amplification bias of our multiplex primers, we amplify the synthetic TCRG template pool with an equimolar mixture of each VF and JR primer, in six PCR replicates. We identify input templates that are over-represented (for example, TCRGVA ), under-represented (for example, TCRGV08 ) and severely under-represented (for example, TCRGV11 ) ( Fig. 4a ). Using an ANOVA, we find that while each JF and VR primer has a characteristic amplification bias, no significant evidence for specific interactions is observed ( P =0.11 by F-test), allowing us to conclude that VF and JR primer amplification biases can be treated independently when adjusting primer concentrations to reduce amplification bias. 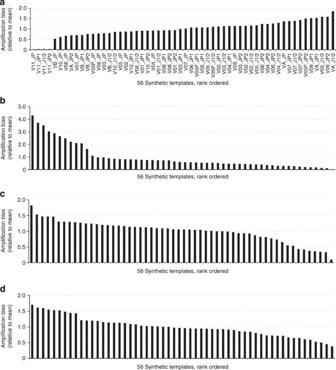Figure 4: Amplification bias across iterative primer mix optimization. The PCR amplification bias (proportional representation, relative to mean) of each of our 56 synthetic templates is calculated for an equimolar mix ofTCRGVF and JR primers (a; in panela, the 56 synthetic templates are rank-ordered and labelled). Subsequent optimizations of primer concentrations produce increasingly better primer mixes (b,c), iterations 1 and 2, with a final primer mix (d) producing the best result. Figure 4: Amplification bias across iterative primer mix optimization. The PCR amplification bias (proportional representation, relative to mean) of each of our 56 synthetic templates is calculated for an equimolar mix of TCRG VF and JR primers ( a ; in panel a , the 56 synthetic templates are rank-ordered and labelled). Subsequent optimizations of primer concentrations produce increasingly better primer mixes ( b , c ), iterations 1 and 2, with a final primer mix ( d ) producing the best result. Full size image Minimizing primer amplification bias and measuring robustness To ensure that each primer is sensitive to changes in concentration, we perform primer titration tests (one VF or JR primer at a time is increased two-fold or four-fold in concentration) to show that increasing the concentration of an individual primer within the PCR mix increases the post-amplification template representation of the targeted templates. However, the magnitude of change varies by primer. We identify one VF primer ( TCRGV11 ) for which increasing concentration does not effectively change the frequency of templates with TCRBV11; we redesign this primer to be more responsive ( Table 1 ). We hypothesize that increasing the concentration of primers that target under-represented gene segments and decreasing the concentration of primers that target over-represented gene segments will reduce the difference between pre- and post-amplification template representation. In our initial experiment (using equimolar VF and JR primers), V11 is highly under-represented, whereas V09 and VA are over-represented; The V01-V08 gene segments, which are all targeted by a single VF primer, show even representation. After eight iterations of altering primer mixes, we create a primer pool that amplifies all 56 synthetic TCRG templates at similar levels ( Fig. 4d ), with a dynamic range of 4.5 (max bias/min bias) and log SS (sum of squared log(amplification bias relative to mean) values) of 1.2, compared with a dynamic range of 104 and log SS of 10 using an equimolar primer mix ( Fig. 4a ). Three independent mixes of this final primer mix have modest levels of variation, indicating that further refinement is limited by the mixing precision of the final primer recipe. Replicate runs using the same lot of primers show highly reproducible results (mean R 2 among three replicates 0.962; Fig. 5 ). Next, we confirm experimentally that the modified primer mix is robust over a 10,000-fold variation in template composition ( Fig. 6 ), allowing for meaningful quantitation of templates at unusually high or low representation in the starting material. Finally, we use highly diverse biological samples to determine that GC content and CDR3 length of sequence between the VF and JR primers have a minimal effect on amplification bias, as expected ( Fig. 7 ). 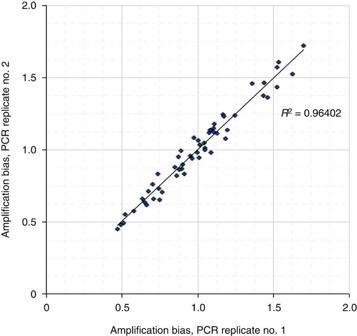Figure 5: Reproducibility of PCR amplification bias. To assess the reproducibility of PCR amplification bias in our multiplex assay, we use our optimized set of TCRG VF and JR primers (iteration 9) to amplify the synthetic reference template input in three replicate PCR reactions. We plot the amplification bias of eachTCRGV/J template from two PCR replicates. Multiplex PCR reactions using the same primer mix generate highly reproducible results (meanR2of 0.962 among three replicate experiments). Figure 5: Reproducibility of PCR amplification bias. To assess the reproducibility of PCR amplification bias in our multiplex assay, we use our optimized set of TCRG VF and JR primers (iteration 9) to amplify the synthetic reference template input in three replicate PCR reactions. We plot the amplification bias of each TCRG V/J template from two PCR replicates. Multiplex PCR reactions using the same primer mix generate highly reproducible results (mean R 2 of 0.962 among three replicate experiments). 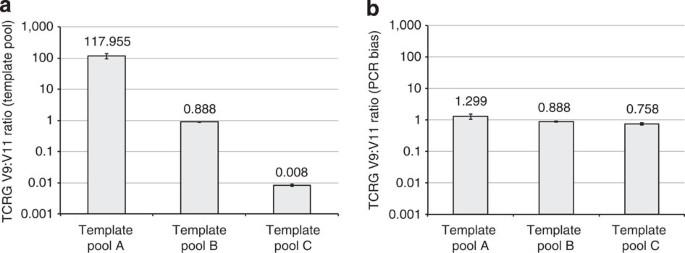Figure 6: Robustness of assay to template concentration. In order to test how stable the relative efficiency of our multiplex PCR approach is across templates which may vary considerably in frequency, we construct three pools of synthetic templates in which the amount of our TCRGV9 and TCRGV11 templates is varied. In the first pool, V9 templates are present at ~100:1 compared with V11 templates; in the second pool all V9 and V11 templates are included at nominally equal concentrations; in the third pool, V9 templates are present at ~1:100 compared with V11 templates. (a) Relative proportions of V9:V11 synthetic templates in the three template pools, as measured by direct sequencing of synthetic template pools. Values are the mean and s.d. of three replicates. (b) Relative ratio of PCR bias between V9 and V11 templates in the three template pools. Values are the mean and s.d. of five replicates. On average we sequence V9 23,000 times and V11 200 times in pool A; V9 12,000 times and V11 14,000 times in pool B; V9 260 times and V11 32,000 times in pool C, which is then corrected according to the known concentrations in the template pool to generate PCR bias values. The relative amplification efficiency of our TCRGV primers is quite robust to changes in template concentration; a small difference is observed in the relative amplification efficiency of V9 and V11 templates (1.7-fold) when these templates’ representation in the PCR starting material is varied over a 10,000-fold range. Full size image Figure 6: Robustness of assay to template concentration. In order to test how stable the relative efficiency of our multiplex PCR approach is across templates which may vary considerably in frequency, we construct three pools of synthetic templates in which the amount of our TCRGV9 and TCRGV11 templates is varied. In the first pool, V9 templates are present at ~100:1 compared with V11 templates; in the second pool all V9 and V11 templates are included at nominally equal concentrations; in the third pool, V9 templates are present at ~1:100 compared with V11 templates. ( a ) Relative proportions of V9:V11 synthetic templates in the three template pools, as measured by direct sequencing of synthetic template pools. Values are the mean and s.d. of three replicates. ( b ) Relative ratio of PCR bias between V9 and V11 templates in the three template pools. Values are the mean and s.d. of five replicates. On average we sequence V9 23,000 times and V11 200 times in pool A; V9 12,000 times and V11 14,000 times in pool B; V9 260 times and V11 32,000 times in pool C, which is then corrected according to the known concentrations in the template pool to generate PCR bias values. The relative amplification efficiency of our TCRGV primers is quite robust to changes in template concentration; a small difference is observed in the relative amplification efficiency of V9 and V11 templates (1.7-fold) when these templates’ representation in the PCR starting material is varied over a 10,000-fold range. 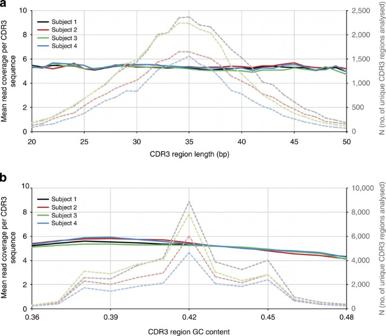Figure 7:TCRGamplification bias by CDR3 region length and GC content. The effect of the length of the CDR3 region and GC content on PCR amplification efficiency by sequencing theTCRGlocus in αβ T cells from four individuals. (a) Mean read coverage as a function of CDR3 length after correcting for amplification bias. (b) Effect of GC content on mean read coverage. In both the panels solid lines represent mean read coverage for each of the four subjects, and dashed lines indicate the number of observations (average of three technical replicates; right axis). Full size image Figure 7: TCRG amplification bias by CDR3 region length and GC content. The effect of the length of the CDR3 region and GC content on PCR amplification efficiency by sequencing the TCRG locus in αβ T cells from four individuals. ( a ) Mean read coverage as a function of CDR3 length after correcting for amplification bias. ( b ) Effect of GC content on mean read coverage. In both the panels solid lines represent mean read coverage for each of the four subjects, and dashed lines indicate the number of observations (average of three technical replicates; right axis). Full size image Computational adjustments to normalize amplification bias Amplification bias factors derived from our final multiplex primer mix using the synthetic template pool allow a straightforward normalization procedure to computationally remove residual amplification bias from libraries amplified using the same multiplex primer mix. We calculate residual scaling factors using the ratio of pre- to post-amplification frequency for each of the 56 templates. Each V or J gene segment is assigned the mean ratio of its constituent templates (that is, for each V segment we calculate the mean amplification bias among the templates using that gene segment) and use these as the final normalization factors to correct sequencing output (that is, the number of reads) for increased accuracy. Assay validation on clinical samples To ensure that our multiplex PCR assay attains high sensitivity and accurate quantitation of biological TCRG rearrangements, we use our optimized assay to amplify and sequence T cells with several different spike-in levels of a cell line bearing a clonal TCRG rearrangement. The results confirm that in a complex biological background, our assay is highly quantitative and sensitive to a level of 1 T cell in 20,000 (1 cell in 100,000 overall; Fig. 8 ). 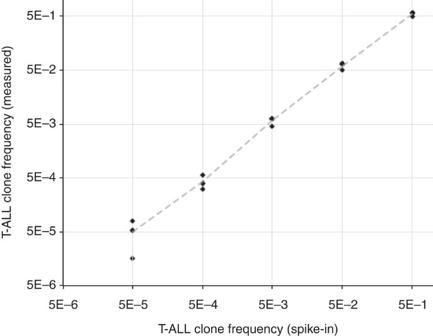Figure 8: Quantitation of T-ALL cells in a complex background. In order to test the ability of our assay to accurately quantitate low levels of targetTCRGsequences in a complex biological background, we create mixtures of gDNA from PBMC and fibroblasts and spike-in gDNA from a clonal population of T cells at five different concentrations ranging from 10 to 0.001% of total cells (50 to 0.005% of T cells). Our multiplex PCR and sequencing assay is run in triplicate for each dilution. Results are shown above, with frequency estimates from our multiplex PCR and sequencing assay presented in triplicate for each spike-in concentration and expected frequency shown in grey. Our assay produces a highly accurate estimate of the proportion of T-ALL gDNA across five orders of magnitude with minimal variance between replicate samples. Figure 8: Quantitation of T-ALL cells in a complex background. In order to test the ability of our assay to accurately quantitate low levels of target TCRG sequences in a complex biological background, we create mixtures of gDNA from PBMC and fibroblasts and spike-in gDNA from a clonal population of T cells at five different concentrations ranging from 10 to 0.001% of total cells (50 to 0.005% of T cells). Our multiplex PCR and sequencing assay is run in triplicate for each dilution. Results are shown above, with frequency estimates from our multiplex PCR and sequencing assay presented in triplicate for each spike-in concentration and expected frequency shown in grey. Our assay produces a highly accurate estimate of the proportion of T-ALL gDNA across five orders of magnitude with minimal variance between replicate samples. Full size image Finally, to test if these assay modifications translate into clinical application, we apply our optimized assay to samples collected from 36 T-ALL patients. For patients with a clonal TCRG rearrangement, we find the frequency of cancer clone concordant between high-throughput sequencing and multi-parameter flow cytometry (mpFC) ( Fig. 9a ). For MRD detection, our assay is concordant with mpFC results, in all cases, with no false-negatives ( Fig. 9a,b ). Further, the PCR-based assay is able to detect MRD in 10 additional patients with a greater detection sensitivity (<10 −5 clone frequency) than mpFC. Quantitatively, the sequencing results are in good agreement with the mpFC data ( Fig. 9a,b ). Most T cells carry two TCRG rearrangements; quantitative detection of MRD by sequencing requires that these two alleles be detected at equal frequency. As would be expected from an unbiased assay, in this experiment both TCRG alleles from each malignant clone are detected at equal frequency in each patient 29 days post-treatment ( R 2 =0.99; Fig. 9c ). 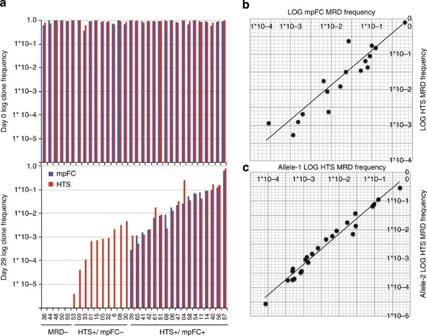Figure 9: Detection of MRD in T-ALL using the optimizedTCRGmultiplex PCR assay (a) T-cell clonality as detected by high-throughput sequencing (HTS) and mpFC. Pre-treatment (top panel) and post-treatment, day 29 (bottom panel) clonal T lymphoblast populations are identified by multiplex PCR and HTS (red) or by mpFC (blue). HTS data are reported as the frequency of the sum of both clonal sequences among total rearranged T-cell sequences; mpFC data are reported as the percentage among total T cells, including all CD7+ T/NK events by mpFC. Based on MRD detection, three groups of cases are identified in post-treatment samples (left to right): (1) no MRD detected (MRD −), (2) MRD detected by HTS, but not by mpFC (HTS MRD +/mpFC MRD −) and (3) MRD detected by both HTS and mpFC (HTS MRD +/mpFC MRD +). (b) MRD frequency as detected by mpFC (xaxis) and HTS (yaxis). For sequencing, MRD frequency is the sum of both alleles. (c) MRD allele frequency of the twoTCRGalleles by HTS in samples with two rearrangements. Figure 9: Detection of MRD in T-ALL using the optimized TCRG multiplex PCR assay ( a ) T-cell clonality as detected by high-throughput sequencing (HTS) and mpFC. Pre-treatment (top panel) and post-treatment, day 29 (bottom panel) clonal T lymphoblast populations are identified by multiplex PCR and HTS (red) or by mpFC (blue). HTS data are reported as the frequency of the sum of both clonal sequences among total rearranged T-cell sequences; mpFC data are reported as the percentage among total T cells, including all CD7+ T/NK events by mpFC. Based on MRD detection, three groups of cases are identified in post-treatment samples (left to right): (1) no MRD detected (MRD −), (2) MRD detected by HTS, but not by mpFC (HTS MRD +/mpFC MRD −) and (3) MRD detected by both HTS and mpFC (HTS MRD +/mpFC MRD +). ( b ) MRD frequency as detected by mpFC ( x axis) and HTS ( y axis). For sequencing, MRD frequency is the sum of both alleles. ( c ) MRD allele frequency of the two TCRG alleles by HTS in samples with two rearrangements. Full size image Multiplex PCR is a general method for targeted, parallel amplification of multiple targets. However, it is difficult to fully optimize multiplex PCR conditions to be precise and quantitative across all target loci [17] . Although it has been generally accepted that multiplex PCR can create significant amplification bias in immune receptor amplification assays [18] , utilizing the recent technological advances in long (~500 bp) oligonucleotide synthesis and high-throughput sequencing our method presents a framework for minimization of PCR amplification bias and additional computational normalization to remove residual bias, resulting in a quantitative readout. We applied this framework to the specific problem of optimizing a multiplex PCR for sequencing TCRG rearrangements in T cells. We synthesized a unique template targeting each possible combination of forward and reverse primers. This synthetic template pool made it possible to exactly quantitate the abundance of each synthetic template pre- and post-multiplex PCR, allowing us to optimize primer concentrations in the multiplex PCR reaction and computationally correct residual bias. Our results have broad potential application in understanding and characterizing the breadth and depth of the immune receptor repertoire as it interacts with pathogens and environmental challenges, and also in haematological oncology where quantitative B- or T-cell cancer clone tracking (that is, minimum residual disease) is needed for patient monitoring and treatment decisions. Previously, the field of immune receptor sequencing has been divided between proponents of gDNA sequencing (which leads to quantitation biased by uneven multiplexed PCR amplification) and cDNA sequencing (which leads to quantitation biased by the imperfect relationship between cell numbers and transcript abundance) [19] . The noise introduced by sequencing cDNA in lieu of gDNA is biological in nature and no artifice will suffice to remove it. The bias introduced by multiplex PCR amplification, however, is purely a product of technical constraints. We demonstrate here that these constraints can be overcome through proper development of a multiplex PCR assay, offering a powerful new method for quantifying and profiling T-cells. Although we describe our method in the context of a multiplex PCR assay for the human TCRG repertoire, the method is generalizable to other adaptive immune receptor loci (for example, IgH, TCRB , TCRA and so on), and should enable the development of any multiplex PCR system where quantitative results are of interest (for example, real-time qPCR). As sequencing of multiplexed libraries (whether B- or T-cell receptors or other targets) moves toward clinical diagnostic applications, the method presented here can serve as a benchmark for unbiased, quantitative multiplex PCR library preparation. Synthetic TCRG template design The human TCRG locus encodes fourteen variable (V) and five joining (J) segments. We created a template mixture of DNA molecules encoding 56 V-J (14 V * 4 J gene) combinations (two J genes ( TCRGJ1 and TCRGJ2 ) were combined due to sequence similarity). A schematic of the synthetic template components is presented in Fig. 1 . Templates were designed to be 495 bases and allow for direct sequencing using either (a) the universal adaptors without multiplex PCR, or (b) the multiplex PCR primer assay we have developed for this locus. Each template included (5′–3′) universal primer UA, a 16 base pair (bp) barcode unique to the specific V/J pair, 300 bp of a V gene extending 5′ from the V segment recombination signal sequence, a second copy of the 16 bp barcode, 100 bp extending 3′ from the J gene recombination signal sequence, a third copy of the barcode and universal primer UB ( Fig. 1 ). The central barcode was also flanked with an in-frame stop codon and a SalI restriction enzyme site, to facilitate computational recognition of this barcode region. The barcodes were selected to be 45–55% GC content, for similar amplification kinetics. The V and J barcodes allowed us to unambiguously identify each template, independent of the actual V and J gene sequence. Templates were, in total, 495 bp and were ordered as double-stranded full-length gBlocks (Integrated DNA Technologies, Coralville, IA). Templates were synthesized and pooled at nominally equimolar levels, and then the relative representation of each template within the pool was measured by high-throughput sequencing of a library prepared by simplex PCR with universal primers UA and UB, tailed with Illumina adaptor sequences for compatibility with the Illumina MiSeq instrument (Illumina, Inc, San Diego, CA, USA). To quantify the composition of the pool, we collected sequence extending from universal primer UB through the first 16 bp barcode of the tailed pool ( Fig. 1a ) and 13 bp into the J gene sequence. Multiplex PCR conditions The multiplex PCR reaction is designed to amplify all possible V and J gene rearrangements of the TCRG locus, as annotated by the IMGT collaboration [20] . The locus includes 14 unique V genes; six functional genes (TCRGV2, 3, 4, 5, 8 and 9 ), three putative open-reading frames lacking critical amino acids for function (TCRGV1, 10 and 11) and five pseudogenes (TCRGV5P, 6, 7, A and B); and five functional J genes. The target sequence for primer annealing was identical for some V segments, permitting amplification of 14 V segments with just 10 unique forward primers. Similarly, four unique reverse primers anneal to all five J genes ( Table 1 ). PCR (25 μl each) were set up at 2.0 μM VF, 2.0 μM JR pool (Integrated DNA Technologies), 1 μM QIAGEN Multiplex Plus PCR master mix (QIAGEN, Valencia, CA, USA), 10% Q- solution (QIAGEN) and 100,000 target molecules from our synthetic TCRG repertoire mix. The following thermal cycling conditions were used in a C100 thermal cycler (Bio-Rad Laboratories, Hercules, CA, USA): one cycle at 95 °C for 6 min, 35 cycles at 95 °C for 30 s, 61 °C for 60 s and 72 °C for 60 s, followed by one cycle at 72 °C for 3 min. For all experiments, each PCR condition was replicated three times unless otherwise noted. Sequencing conditions To quantify the composition of the synthetic TCRG template pool, simplex low-cycle PCR libraries were sequenced for a total of 29 bases from the universal primer UB on an Illumina MiSeq (Illumina), extending across the third 16 bp barcode, to identify the synthetic molecule, and 13 bases into the J gene, to ensure specificity ( Fig. 1b ). These data precisely measured the composition of the synthetic TCRG repertoire before multiplex PCR. To assess amplification bias of the multiplex PCR reaction, we sequenced 58 bases of the template. For sequencing, we used primers specific to the J gene and sequenced the remaining 15 bases of the J gene and 25 bases of the stop codon, second barcode, and the restriction enzyme site, and 17 bases of the V gene. Barcode frequencies from the multiplex PCR library were compared with frequencies observed in the simplex PCR library, to determine relative bias in amplification of each template. In later experiments involving biological templates, we sequenced 78 bases from the JR segment-specific primers, in order to identify both the V and J segments uniquely, and to precisely measure the length and GC content of the CDR3 region. Primer mix optimization Following initial bias assessment, we performed experiments to define individual primer amplification characteristics. In order to determine the specificity of our VF and JR primers, we prepared 10 mixtures containing a single VF primer with all JR primers, and 4 mixtures containing a single JR primer with all VF primers. We used these primer sets to amplify the synthetic templates and sequenced the resulting libraries to measure the specificity of each primer for the targeted V or J gene segments and to identify instances of off-target priming. Titration experiments were performed using pools of two-fold and four-fold concentrations of each individual VF or JF within the context of all other equimolar primers (for example, 2x-fold TCRGV09+all other equimolar VF and JR primers) to allow us to estimate scaling factors relating primer concentration to observed template frequency. Using the scaling factors derived by titrating primers one at a time, we developed alternative primer mixes in which the primers were combined at uneven concentrations to minimize amplification bias. The revised primer mixes were then used to amplify the template pool and measure the residual amplification bias. We iterated this process, reducing or increasing each primer concentration appropriately based on whether templates amplified by that primer were over or under-represented in the previous round of results. At each stage of this iterative process, we determined the overall degree of amplification bias by calculating two metrics based on the amplification bias (relative to mean) of each template: dynamic range (max bias/min bias) and sum of squared log(bias) values; we iterated the process of adjusting primer concentrations until there was no improvement between iterations. Robustness of assay to template concentration To assess the robustness of the final optimized primer mix and scaling factors to deviations from equimolar template input, we used a highly uneven mixture of TCRG reference templates to determine the effect on sequencing output. We generated three different mixtures of the TCRG reference templates. Template pool A was mixed to be have an abundance of V9 templates, a template amplified by an over-amplifying primer, and a minimal number of V11 templates, a template amplified by an under-amplifying primer (at a ratio of ~100:1). Template pool B was mixed to include all templates at even concentrations. Template pool C was mixed to have an abundance of V11 templates and minimal number of V9 templates (at a ratio of ~100:1). These templates mixes were quantified and then amplified with our adjusted primer mix. Robustness to variable region sequence characteristics Our standardized TCRG templates are identical in length for all V/J pairs, and have very similar GC content. We sequenced sorted αβ T cells from four healthy individuals, to test for the effect of GC content and/or CDR3 length on amplification bias using the final optimized primer set. We amplified TCRG rearrangements from biological samples (three replicates each) of sorted αβ T cells (~40,000) from four healthy adult subjects. Specifically, we evaluated the effect of GC content and/or CDR3 length on PCR amplification bias. Both TCRG alleles are rearranged in αβ T cells [8] , however, αβ T-cell selection is not related to the TCRG locus rearrangement. This property makes αβ T cells an ideal sample source to test these sequence context effects. To reduce noise introduced by large clonal expansions, sequences observed more than 10 times in the data were discarded. After computationally adjusting for residual amplification bias attributable to the specific VF and JR primers, we compared the sequencing read depth achieved for each TCRG rearrangement with its GC content and CDR3 length. An average of 28,000 such TCRG rearrangements were observed in each patient. Quantitation of T-ALL cells in a complex background In order to test the sensitivity, reproducibility and quantitative accuracy of our method on biological rather than synthetic templates, we created a mixture of 10% gDNA from clonal T-ALL cells (Coriell no. NA02219), 10% gDNA from a healthy adult’s PBMC and 80% fibroblast gDNA. This original DNA mixture was serially diluted to create mixtures with the following overall proportions of T-ALL gDNA: 10%, 1%, 0.1%, 0.01%, 0.001%. Our multiplex PCR and sequencing assay was run in triplicate for each dilution. Detection of MRD in clinical samples To test if the optimized assay would translate into clinical testing, we assayed samples collected from 36 T-ALL patients enrolled in the Children’s Oncology Group AALL0434 trial. All samples were de-identified before using our TCRG assay. All patients provided informed consent as part of the COG trial for the use of their residual samples. Samples from two time points were tested: before induction therapy (day 0), and 29 days following induction therapy (day 29). Samples were submitted for mpFC analysis at University of Washington as part of the AALL0434 COG trial protocol. Residual bone marrow from each patient was obtained for sequencing following mpFC analysis. Samples were processed for mpFC using standard methods for surface (tube 1; NH 4 Cl+0.25% formaldehyde) or surface and cytoplasmic (tube 2; Fix and Perm (Invitrogen)) antigens, and 750,000 events acquired on a Becton-Dickinson LSRII. Clusters of events that differed from normal T-cell maturation were designated MRD and quantified relative to total mononuclear cells and CD7+ T/NK cells. Data were analysed using Woodlist software version 2.7. These data were used to estimate the frequency of blast cells and CD7+ cells (T cells) in each sample. As previously described, using TCRG sequencing we identified one or two dominant CDR3 sequences in the pre-treatment sample (which are presumed to be the TCRG rearrangements in the malignant clone) and determined MRD status based on the presence of those sequences in the post-treatment sample [9] . We compared the frequency of the top cancer clone in each patient to the results obtained by mpFC. To assess whether the detection variation was due to sequencing bias, we utilized only the data from 32 patients with both TCRG alleles rearranged and compared the frequency with the paired alleles. How to cite this article: Carlson, C. S. et al . Using synthetic templates to design an unbiased multiplex PCR assay. Nat. Commun. 4:2680 doi: 10.1038/ncomms3680 (2013).